A strong electro-optically active lead-free ferroelectric integrated on silicon The development of silicon photonics could greatly benefit from the linear electro-optical properties, absent in bulk silicon, of ferroelectric oxides, as a novel way to seamlessly connect the electrical and optical domain. Of all oxides, barium titanate exhibits one of the largest linear electro-optical coefficients, which has however not yet been explored for thin films on silicon. Here we report on the electro-optical properties of thin barium titanate films epitaxially grown on silicon substrates. We extract a large effective Pockels coefficient of r eff =148 pm V −1 , which is five times larger than in the current standard material for electro-optical devices, lithium niobate. We also reveal the tensor nature of the electro-optical properties, as necessary for properly designing future devices, and furthermore unambiguously demonstrate the presence of ferroelectricity. The integration of electro-optical active films on silicon could pave the way towards power-efficient, ultra-compact integrated devices, such as modulators, tuning elements and bistable switches. The presence of functional properties in many perovskite materials [1] , [2] has pushed the development of integrating such crystals directly on silicon (Si) to realize a variety of new devices [3] . Since the first methods to epitaxially deposit perovskite thin films on Si were established [4] , the growth process has been carefully optimized [5] and single crystalline layers were fabricated even on large-scale 8′′ substrates [6] . However, the interest in this research field has mainly been motivated by the use of oxides in the electronic domain, such as memory applications [7] , gate dielectrics in field-effect transistors [8] or all-oxide electronics [9] . Meanwhile, the steadily improving performance of complementary metal oxide semiconductor (CMOS) technology increases the difficulty to handle inter- or intra-chip data communication by means of electrical wiring [10] because of power constraints in combination with increased bandwidth demands. In this context, devices working in the optical domain have emerged as a mature field of research [11] , and building blocks required for a functional photonic network such as detectors [12] or modulators [13] have already been integrated on Si. However, today’s silicon photonics technology does not exploit the linear electro-optical (EO) properties available in oxides, which for decades fuelled the progress in telecommunication based on fibre optics to extremely high modulation speeds with well-established devices [14] . In recent work, micro-scale EO devices have been presented [15] . These devices were based on LNO (LiNbO 3 ), which can be integrated as high-quality films on Si only via complex and costly layer-bonding approaches [16] . On the other hand, a non-vanishing Pockels effect has also been reported directly in Si, by exploiting strain effects that break the crystalline symmetry [17] , [18] . However, these approaches are both limited to relatively small EO coefficients ( r LNO ≈30 pm V −1 (ref. 14 ), r Si ≈1.7 pm V −1 (ref. 18 ) compared with those of alternative oxides (for example, barium titanate (BTO), r BTO >1,000 pm V −1 ) (ref. 19 ), which drastically narrows the range of potential applications. Our work demonstrates that large Pockels coefficient can be obtained in high-quality oxide thin films epitaxially grown on Si. This enables a flexible way to develop novel devices in silicon photonic circuits that benefit from the established EO know-how of fibre optics. BTO (BaTiO 3 ) is the material of choice because of its strong EO properties in bulk form, the earlier demonstration of EO devices using BTO thin films on oxide substrates [20] , [21] , and its compliance with possible future regulations excluding lead from products. Additionally, bulk BTO is a ferroelectric, which is an appealing class of materials for bistable electrical and optical applications. This ferroelectric behaviour is, as shown in our study, maintained even in thin films. Film growth and structural characterization The EO properties of BTO are tightly connected with its crystalline structure, which is described in a non-centrosymmetric tetragonal P 4 mm space group compatible with a non-vanishing linear Pockels effect [22] . Although the tetragonal phase is stable in bulk BTO crystals at room temperature, polycrystalline BTO thin films tend to stabilize in a cubic symmetry [23] , which originates from the formation of small grains, without Pockels effect. We suppressed such grain formation by depositing our 130-nm-thick BTO film epitaxially on a Si substrate covered by a 4-nm-thin strontium titanate (STO) buffer layer. Out-of-plane and grazing-incidence in-plane X-ray diffraction (XRD) measurements ( Fig. 1a ) confirmed the epitaxial relationship and showed that the crystal symmetry is tetragonal with its long tetragonal c -axis parallel to the sample surface. While an out-of-plane oriented c -axis can be obtained by growing highly compressively strained films, for example by reducing their thickness, an in-plane-oriented c -axis is expected in our thick films that are fully relaxed at the growth temperature. This orientation, which has to be considered carefully when interpreting any EO response, results from biaxial tensile strain after cooling, due to the different thermal expansion coefficients of BTO and Si (ref. 24 ). As the template for the epitaxial growth is a cubic Si substrate, two equivalent orientations of the elongated tetragonal c -axis exist. By forming domains in which the c -axis is rotated by 90° within the plane of the film, strain fields originating from the mismatch between the cubic Si and tetragonal BTO lattice are compensated. The existence of two orthogonal domains is evidenced by the presence of the convoluted [200] BTO and [002] BTO diffraction peaks in the grazing-incidence XRD data ( Fig. 1a , inset). As no intentional miscut was present in the substrate, the population ratio of these domains is assumed to be 1:1 for symmetry reasons. The epitaxial relationship between BTO, STO and Si is visualized in high-resolution scanning transmission electron microscopy (STEM) analysis ( Fig. 1b , left). Low-resolution images reveal that defects in the BTO develop mainly perpendicularly to the interface ( Fig. 1b , right), likely because of strain compensation at the interfaces of orthogonal domains. From both XRD and STEM analyses we infer that the different domains penetrate the film to form a structure as shown in Fig. 1c . The arrows indicate the spontaneous polarization present in tetragonal BTO along the crystalline c -axis. This ferroelectric structure of the film is critical for the EO analysis presented here. 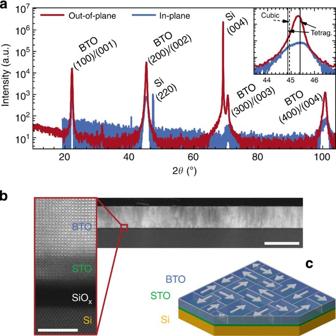Figure 1: Structural analysis. (a) XRD diagram of 130 nm BTO on 4 nm STO on Si; the inset shows a magnification of the BTO (200)/(002) peak obtained with out-of-plane and in-plane geometries. The vertical lines correspond to bulk values of tetragonal (solid) and cubic (dashed) BTO (ref.35). (b) Cross-sectional high-angle annular dark-field STEM image of the interface region showing Si, SiOx, STO and BTO (scale bar, 5 nm), and a corresponding low-magnification cross-section of the sample in dark-field mode (scale bar, 200 nm). The red square indicates the area from which the high-resolution micrograph was recorded. Defects penetrate mainly perpendicularly to the interface. (c) Schematic of the domain structure in the BTO film with randomly oriented spontaneous polarization associated with thec-axis direction (white arrows in blue cuboids). a.u., arbitrary unit. Figure 1: Structural analysis. ( a ) XRD diagram of 130 nm BTO on 4 nm STO on Si; the inset shows a magnification of the BTO (200)/(002) peak obtained with out-of-plane and in-plane geometries. The vertical lines correspond to bulk values of tetragonal (solid) and cubic (dashed) BTO (ref. 35 ). ( b ) Cross-sectional high-angle annular dark-field STEM image of the interface region showing Si, SiO x , STO and BTO (scale bar, 5 nm), and a corresponding low-magnification cross-section of the sample in dark-field mode (scale bar, 200 nm). The red square indicates the area from which the high-resolution micrograph was recorded. Defects penetrate mainly perpendicularly to the interface. ( c ) Schematic of the domain structure in the BTO film with randomly oriented spontaneous polarization associated with the c -axis direction (white arrows in blue cuboids). a.u., arbitrary unit. Full size image Qualitative determination of Pockels effect The EO characterization was performed at the standard telecom wavelength of λ=1.55 μm, which is compatible with the silicon photonic technology. The EO properties of the film were determined by investigating the polarization changes of a laser beam transmitted between a pair of electrodes separated by a small, micrometre-scale gap. Applying a potential difference between two electrodes results in an electric field E within the gap, modifying the refractive index n ( E ) of BTO (ref. 21 ) In this simplified equation that neglects any tensor properties [19] , r is the Pockels coefficient and n 0 the refractive index when no electric field is applied. To gain sensitivity by using a lock-in detection scheme, the applied voltage is modulated by V a.c. =3 V (peak-to-peak) at a frequency of f =17.3 kHz around a d.c. offset voltage V off =25 V, which is sufficiently high to align the ferroelectric domains. The modification of the refractive index due to the applied field leads to a rotation of the linear polarization of the transmitted beam by an angle δ ( Fig. 2a ). After passing through an analyzer oriented at an angle θ a relative to the polarization of the incident beam, the transmitted power P ~cos 2 ( θ a − δ ) (ref. 19 ) depends on the induced rotation of the polarization. For small angles δ , the power variations are expected to be proportional to the derivative d P/ d θ a (ref. 25 ). The measured response of our sample is in excellent agreement with such a dependence ( Fig. 2b ), confirming the existence of an EO effect. We can rule out a varying absorption as the origin of the power modulation Δ P because in that case, Δ P would be proportional to the absolute transmitted power, in contrast to the observed EO response. The linear dependence of Δ P on the applied field ( Fig. 2b , inset) further precludes the quadratic EO Kerr effect to be dominant and thus confirms the presence of the linear Pockels effect in our sample. 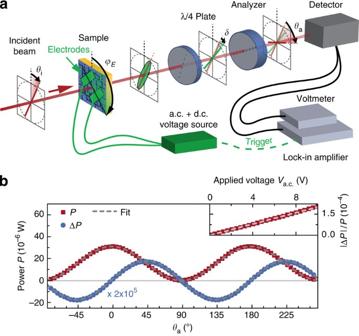Figure 2: Principle of EO characterization. (a) Schematics of measurement setup indicating the variation of the polarization states when an electric field (green) is applied by an a.c./d.c. voltage source.φEis the angle between the BTO [h00] and [00h] crystallographic axes and the applied electric fieldE. The small rotationδof the polarization results in a modulation of the transmitted power at the detector, which is recorded with a lock-in amplifier. (b) Transmitted powerPand variation in power ΔPdue to the EO effect as a function of the analyzer positionθa, taken forθi=0° across a 17-μm-wide gap oriented atφE=45° with an applied voltage offset ofVoff=25 V. Inset inbshows the normalized linear power change |ΔP|/Patθa=45° andVoff=25 V as a function of the peak-to-peak amplitudeVa.c.. Figure 2: Principle of EO characterization. ( a ) Schematics of measurement setup indicating the variation of the polarization states when an electric field (green) is applied by an a.c./d.c. voltage source. φ E is the angle between the BTO [h00] and [00h] crystallographic axes and the applied electric field E . The small rotation δ of the polarization results in a modulation of the transmitted power at the detector, which is recorded with a lock-in amplifier. ( b ) Transmitted power P and variation in power Δ P due to the EO effect as a function of the analyzer position θ a , taken for θ i =0° across a 17-μm-wide gap oriented at φ E =45° with an applied voltage offset of V off =25 V. Inset in b shows the normalized linear power change |Δ P| / P at θ a =45° and V off =25 V as a function of the peak-to-peak amplitude V a.c. . Full size image Dependence of EO response on measurement geometry To further explore the tensor nature of the Pockels effect [19] , the dependence of δ on the angle between the applied electric field, incident polarization, and crystallographic orientation has to be considered carefully. The derivation of a field-normalized angle δ′ from data sets, as shown in Fig. 2 , is described in the Methods section. In general, applying an electric field to an anisotropic material with a linear EO effect results in a change of the birefringence Δ n by Δ(Δ n ) and a rotation of the optical axis by Δ γ ( Fig. 3a ). In our measurement geometry, both effects cause a rotation of the polarization of the transmitted beam, but the magnitude of δ′ depends on the incident polarization: If Δ γ is dominant, δ′ is maximal when the incident polarization is parallel to the optical axis of the crystal ( θ i =0°), which is experimentally observed when the applied electric field E is oriented along the [101] BTO direction ( Fig. 3b ). If Δ(Δ n ) is dominant, on the other hand, δ′ is maximal for | θ i |~45°. We also observe this regime in our measurements, when the E is oriented along the [001] BTO /[100] BTO axes. By modelling the EO response of BTO for a single domain [25] ( Fig. 3b , inset), the rotation of its optical axis is predicted to vanish when E is parallel to [001] BTO ( E ||[001] BTO ), whereas a change in the birefringence remains. In contrast, a strongly enhanced rotation of the optical axis is expected for E ||[101] BTO . Both features of the model agree well with our experimental results. The dependence of the EO response on the orientation of the electrodes also precludes any polarization-dependent absorption effect from the edges of the metallic pads. Such effect would be independent of the orientation of the electrodes with respect to the BTO crystalline axis, which is in contrast to the data shown in Fig. 3 . 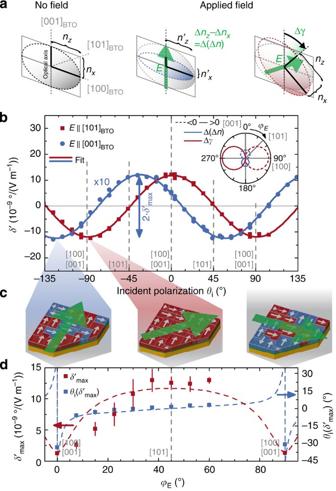Figure 3: Experimental and simulated EO response. (a) Refractive index ellipse in BTO, showing the refractive indexnxandnzalong different crystalline directions (left). Applying an electric fieldEchanges the birefringence Δ(Δn) (centre) and rotates the optical axis (right) depending on the orientation ofE(not to scale). (b) Field-normalizedδ′as function of the angle of incident polarization for two orientations of the applied fieldE. The dashed vertical lines correspond to the main BTO crystalline directions. The inset shows the simulated birefringence change Δ(Δn) and the angle of the optical axis Δγin BTO in arbitrary units. (c) Schematics indicating the different ferroelectric domain configurations for various orientations ofE(green), with domains oriented towards the field (red) and randomly oriented ones (blue). (d) Maximum rotation angleδ′maxand corresponding angle of incident polarizationθi(δ′max) for various values ofφE. The error bars show the standard deviation from several measurements on different electrode pads. The simulated curves (dashed lines) are based on the Pockels tensor that was experimentally determined (details inSupplementary Note 2). Figure 3: Experimental and simulated EO response. ( a ) Refractive index ellipse in BTO, showing the refractive index n x and n z along different crystalline directions (left). Applying an electric field E changes the birefringence Δ(Δ n ) (centre) and rotates the optical axis (right) depending on the orientation of E (not to scale). ( b ) Field-normalized δ′ as function of the angle of incident polarization for two orientations of the applied field E . The dashed vertical lines correspond to the main BTO crystalline directions. The inset shows the simulated birefringence change Δ(Δ n ) and the angle of the optical axis Δ γ in BTO in arbitrary units. ( c ) Schematics indicating the different ferroelectric domain configurations for various orientations of E (green), with domains oriented towards the field (red) and randomly oriented ones (blue). ( d ) Maximum rotation angle δ′ max and corresponding angle of incident polarization θ i ( δ′ max ) for various values of φ E . The error bars show the standard deviation from several measurements on different electrode pads. The simulated curves (dashed lines) are based on the Pockels tensor that was experimentally determined (details in Supplementary Note 2 ). Full size image Ferroelectric properties of the BTO film To quantify the elements of the Pockels tensor, one must take into account not only a single domain but the overall ferroelectric domain structure of the BTO film ( Fig. 1c ): because of the anti-centrosymmetry of the Δ(Δ n ) and Δ γ functions ( Fig. 3b , inset), the induced rotation of the polarization by δ′ will be reversed for a domain that is rotated by 180° and exposed to the identical electric field. The EO response of two anti-parallel domains will thus cancel out. However, anti-parallel domain pairs can be eliminated by flipping their polarization when the applied electric field component E [001] along the crystallographic [001] BTO axis is above the coercive field E c . Hence, a ferroelectric hysteresis loop would be expected in the optical measurements of δ′ on varying the offset of the applied electric field E off . This is indeed observed experimentally ( Fig. 4 ). As expected, the random domain orientation after heating the sample above the Curie temperature of BTO ( T c =124 °C (ref. 26 )) initially shows no EO response at E off =0. By increasing E off , a strong enhancement in δ′ is visible, resulting from the switching of the ferroelectric domains, which eliminates anti-parallel domains. The hysteresis loop monitored during the sweep of E off ( Fig. 4 ) is a clear signature of the ferroelectric nature of the film. Once poled, the ferroelectric domain structure remains stable for several days at least, as can be seen from the small relaxation of the remanent EO response ( Fig. 4 , inset). From the shape of the hysteresis, a coercive field of E c =5 × 10 5 V m −1 is extracted, which is an order of magnitude larger than in bulk BTO. Such an increase is typically observed for ferroelectric thin films because of domain pinning and finite depolarization fields [27] . 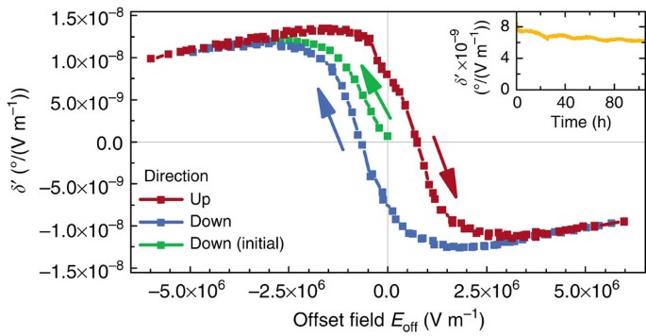Figure 4: Optical response as a function of the offset fieldEoff. The data set is collected in three successive loops measured at 25 °C after heating the film above its bulk Curie temperature (green) and sweepingEoffup (red) and down (blue) again. The finite slope at large |Eoff| values results from nonlinear EO effects. The inset shows the relaxation of the remanentδ′value at room temperature. Figure 4: Optical response as a function of the offset field E off . The data set is collected in three successive loops measured at 25 °C after heating the film above its bulk Curie temperature (green) and sweeping E off up (red) and down (blue) again. The finite slope at large | E off | values results from nonlinear EO effects. The inset shows the relaxation of the remanent δ′ value at room temperature. Full size image The hysteresis in the optical signal qualitatively excludes any influences from the Si-substrate on the EO response of the sample. As recently shown, non-vanishing Pockels coefficients are induced in Silicon if strain-gradients are present [18] , [28] . However, Si remains non-ferroelectric and thus no effects of poling are visible, in clear contrast to our observations. From the measurements shown in Fig. 4 we can furthermore exclude that ferroelectric domain switching [29] has a significant contribution on the EO response presented in Figs 2 and 3 . These measurements were performed in the saturation regime of the hysteresis loop (| E off |>3 × 10 6 V m −1 , see Methods section). The saturation indicates that small changes in the applied field hardly change the domain population. Therefore, the modulation of the electric field by E a.c. =±0.2 × 10 6 V m −1 « E off (Methods section) for the lock-in detection induces only a negligible error in the determination of δ′ and thus of the EO constants. More generally, if domain switching contributed to the EO response, a strong enhancement of δ′ for the regime of | E off + E a.c. |< E c would be expected, because the relative change of the domain population is the strongest for small electric offset fields. This behaviour would also be expected for the unpoled sample and is contrary to our observations of a vanishing EO signal in that regime ( Fig. 4 ), thus excluding domain switching to be a major contribution to δ′ . We can also utilize the hysteresis behaviour for the quantitative determination of the EO constants: indeed, because the offset in the electric field E applied during the measurements ( Fig. 3b ) was significantly above the coercive field, we assume the ferroelectric domains to be aligned to the electric field component E [001] . Domains orthogonal to E experience no component along their long [001] axis, thus keep their anti-parallel configuration ( Fig. 3c ) without any net contribution to the EO response. Taking these domain structures into account, we can calculate the individual components of the reduced 6 × 3 Pockels tensor r (ref. 19 ), which reduces to only three different elements for the P 4 mm symmetry class of tetragonal BTO (ref. 22 ). For E ||[001] BTO , the optical properties are determined by r 13 and r 33 . Considering δ ~ r c = r 33 ( n eo / n o ) 3 r 13 , we obtain r c =30 pm V −1 as the c -axis Pockels coefficient. This r c value [19] is more important for the performance of EO devices than the individual components r 13 and r 33 (ref. 20 ), which are correlated and cannot be independently determined in our measurement geometry. The third tensor element, r 42 , describes the rotation of the optical axis as observed at E ||[101] BTO . A detailed analysis allows us to extract r 42 =105 pm V −1 (see Supplementary Note 1 ). For comparison with previous work [21] , [30] , we calculated an effective value r eff =148 pm V −1 by neglecting the tensor nature of r and simply considering the field-induced phase shift between two orthogonal components of the transmitted light, as described in the Methods section. Our results represent a major improvement compared with the limited number of published data on EO properties of lead-free oxides integrated on silicon [31] , [32] , [33] . The Pockels tensor and our model with multiple domains are validated by systematically varying the orientation of the applied electric field and comparing the experimental results with simulations using the previously determined values for r ( Fig. 3d , more details in the Supplementary Note 2 ). When the electric field is oriented close to the [101] BTO orientation, the EO response originates from a rotation of the optical axis ( θ i ~0°), and the magnitude of the response approaches a maximum. These characteristics are expected for a large r 42 coefficient when the electric field is not parallel to the [001] BTO direction ( Fig. 3b , inset). The situation is reversed when E is aligned to the [001] BTO and [100] BTO axes: The EO response is minimal and determined by the change in birefringence (| θ i |~45°) rather than by the rotation of the optical axis, in excellent agreement with the simulation. Finally, the identical EO response when rotating the electric field by 90° matches the picture of equally distributed orthogonal domains inferred from the structural characterization ( Fig. 1c ). Thus, the Pockels tensor and domain structure derived in our study are consistent with the experimentally observed EO behaviour for various orientations of the applied electric field. In conclusion, we have shown the direct integration of a ferroelectric BTO film on silicon exhibiting a strong linear EO effect with an effective Pockels coefficient of r eff =148 pm V −1 . This value exceeds previous data reported for integrated LNO by at least a factor of five, and for strained Si by a factor of 100. By combining EO measurements with EO simulations, we developed a method to investigate the tensor nature of the Pockels effect of multi-domain thin films, which is essential for properly designing future optical devices. The strong EO response renders the films perfectly suitable as base material for novel applications in the domain of silicon photonics such as tuning or bistable switching. The latter application is especially appealing because of the long remanence demonstrated in the films, which also makes BTO layers attractive for transistors with ferroelectric gates and similar application in the electronic domain. Besides the new opportunities for engineering photonic circuits, the integration of functional oxides such as BTO also opens exciting challenges for material scientists to tailor the EO properties of those oxides by strain engineering or fabrication of superlattice structures [34] , which could ultimately lead to another boost of their EO properties. Sample preparation The sample was prepared in a molecular beam epitaxy chamber with a base pressure of 5 × 10 −10 mbar. A 4-nm-thick STO (SrTiO 3 ) film was deposited on a high-resistive, 500-μm-thick Si(001) substrate using a similar process as described in ref. 8 . It serves as epitaxial seed layer for the subsequent 130-nm-thick BTO layer, which was grown by alternate exposure to Ba and Ti fluxes in atomic oxygen at a pressure of 10 −5 mbar and a temperature of 650 °C. The Ba and Ti fluxes were calibrated with a quartz microbalance. An interfacial SiO x layer can develop during the BTO growth step because of the combination of high temperature and high oxygen pressure, but does not disrupt the epitaxial relationship between Si, STO and BTO as this relationship is established during the initial growth of STO on Si. After the growth, the backside of the wafer was polished for optical transmission measurements. The film thickness was determined by spectroscopic ellipsometry (Woollam VASE). Electrode pairs of 300 nm Pt/10 nm Ti with varying orientation between the BTO crystallographic axes and the electrode gap (0°–90°) with an accuracy of ±1° were fabricated on the samples using standard optical lithography techniques. Unless stated differently, the optical measurements were performed on devices with electrodes having a gap size of ~7 μm. X-ray analysis XRD measurements were carried out on a Bruker Discovery D8 system equipped with a rotating anode generator. A symmetric Ge[220] 4-bounce monochromator was used on the primary beam for the out-of-plane measurements, together with a slit on the diffracted beam. To have a sufficiently high signal-to-noise ratio, grazing-incidence in-plane measurements were performed without monochromator, and using Soller slits on the detector side. By neglecting a possible orthorhombic distortion that would be within the error bars of the XRD data, the lattice parameters of the tetragonal unit cell were determined to be a =3.997±0.005 Å and c =4.032±0.005 Å using the out-of-plane diffraction peaks and by deconvoluting the peaks measured in grazing-incidence in-plane geometry. Transmission electron microscopy Cross-section samples for transmission electron microscopy were cut parallel to the (110) planes of the Si substrate and mechanically polished to a thickness of about 20 μm, followed by final ion milling under grazing incidence until electron transparency was reached. High-angle annular dark-field STEM was carried out using a conventional JEOL 2200FS TEM/STEM microscope operated at 200 kV. The probe semi-convergence angle was set to 10.8 mrad and the inner semi-detection angle of the annular dark-field detector was 100 mrad. EO measurements For the EO characterization (schematics in Fig. 2a , for more details see Supplementary Fig. S1 ), a single-mode diode laser from New Focus operating at λ ≈1.55 μm was first polarized with a Glan-laser prism (extinction ratio <5 × 10 −6 ). A successive half-wave plate mounted on a motorized stage (Newport URS50BPP) was used to set the incident polarization, before focusing the beam with a spot size of ~15 μm into the gap of two electrodes. Owing to the birefringence of BTO, the transmitted light is generally slightly elliptically polarized. A quarter-wave plate after the sample and a second Glan-laser prism, both mounted on motorized stages, were iteratively rotated to minimize the power of the transmitted light on an InGaAs detector. For the condition of minimal transmission, the light polarization after the quarter-wave plate is linear. After applying a voltage offset of V off =40 V for ~1 min to align the ferroelectric domains, a sinusoidal, alternating voltage of V a.c. =3.0 V (peak-to-peak amplitude) at f =17.3 kHz with V off =25 V was applied during the measurements. No electrical breakdown was observed for these voltages (see I – V curve, Supplementary Fig. S2 ). The transmitted power P and the power variations Δ P were recorded using a lock-in amplifier while rotating the analyzer θ a in small steps. The rotation δ was determined by fitting the signal Δ P / P using Δ P = δ × d P /d θ a + A P . In this equation, P ~cos 2 ( θ a − δ )≈cos 2 θ a corresponds to the transmission between two polarizers [19] , and A to background contributions, which are proportional to the transmitted power and caused by interference effects between the domains. With this fitting procedure, a rotation in the polarization down to δ =10 −5 ° can be detected, which is significantly better than the mechanical resolution of the rotation stages . δ was field-normalized by the amplitude of the applied a.c.-field E a.c. , δ′ = δ/E a.c. The magnitude of the applied electric field E is calculated by approximating the field in the gap of width d by E = V d −1 . The Pockels coefficient r c is determined at φ E =0° by r c =Γ λ /(π n 3 E a.c. d ν ) (ref. 30 ), where Γ=2 × δ max is the induced phase shift in the sample and ν =0.5 is the relative volume fraction of the domains parallel to the electric field, which contribute to the EO response. δ max corresponds to the maximum rotation angle when varying the incident polarization ( Fig. 3b ). The effective Pockels coefficient r eff is calculated at φ E =45° in the same way using ν =1. Before measuring the hysteresis loops, the sample was heated to 250 °C for ~10 min to ensure a depolarized domain state in the sample, and then cooled down to room temperature. Each data point during the hysteresis measurement corresponds to a sweep in θ a , taking ~5 min, which yields a typical duration of ~5 h for the measurement of one loop. EO simulations The calculation is based on an algorithm described in ref. 25 using the ordinary and extraordinary refractive indices of bulk BTO ( n o =2.268 and n eo =2.297 at λ =1,550 nm). The EO properties of BTO thin films are typically reduced by an order of magnitude [20] , [21] compared with bulk values ( r 13 =8, r 33 =80, r 42 =1,000 pm V −1 at λ=1,500 nm) (ref. 22 ). Therefore, the bulk values were scaled by a factor of 0.1 in our simulations, resulting in a good qualitative agreement of the simulated EO response with our experimental results. How to cite this article: Abel, S. et al . A strong electro-optically active lead-free ferroelectric integrated on silicon. Nat. Commun. 4:1671 doi:10.1038/ncomms2695 (2013).